The dynamic surface tension of atmospheric aerosol surfactants reveals new aspects of cloud activation The activation of aerosol particles into cloud droplets in the Earth’s atmosphere is both a key process for the climate budget and a main source of uncertainty. Its investigation is facing major experimental challenges, as no technique can measure the main driving parameters, the Raoult’s term and surface tension, σ , for sub-micron atmospheric particles. In addition, the surfactant fraction of atmospheric aerosols could not be isolated until recently. Here we present the first dynamic investigation of the total surfactant fraction of atmospheric aerosols, evidencing adsorption barriers that limit their gradient (partitioning) in particles and should enhance their cloud-forming efficiency compared with current models. The results also show that the equilibration time of surfactants in sub-micron atmospheric particles should be beyond the detection of most on-line instruments. Such instrumental and theoretical shortcomings would be consistent with atmospheric and laboratory observations and could have limited the understanding of cloud activation until now. The activation of aerosol particles into cloud droplets in the atmosphere is generally assumed to be described by the Köhler theory [1] , which involves only two parameters, the surface tension of the forming droplet, σ (mN m −1 ), and the Raoult’s term describing the surrounding water vapour. However, this simple theory is facing major experimental challenges, as today there is no technique able to measure these parameters for the micron or sub-micron particles that are relevant in the atmosphere. The instruments built to investigate these processes, hygroscopicity tandem differential mobility analysers (HTDMA) and cloud condensation nuclei counters (CCNC), do not measure these parameters but indirectly related quantities such as the number or growth of nucleated droplets [2] , [3] , thereby making comparisons between measurements and theory difficult. Another difficulty was that, until recently, the surface tension of atmospheric aerosols could not be measured directly and only specific surface-active compounds, such as humic-like substances [4] , [5] , [6] or sub-fractions [7] , were isolated, thus providing limited information. Thus, while the Köhler theory implies that by lowering the surface tension of atmospheric particles, surfactants should favour their activation into cloud droplets, partitioning models predict that this effect should be largely compensated by the strong surface/bulk concentration gradient of these compounds, also called partitioning [8] , [9] , [10] , [11] . However, recent atmospheric [7] , [12] , [13] and laboratory [14] observations have reported an enhancement of cloud activation due to surfactants, implying that these models and most measurements might be incomplete. In the last few years, an extraction method was developed to isolate the total surfactant fraction of atmospheric particles, thus allowing, for the first time, to study it directly [15] , [16] . The first results have shown that these fractions are much more surface-active than expected ( σ ≤30 mN m −1 ) and display properties similar to those of biosurfactants such as surfactin or rhamnolipids [17] , [18] . Here we present the first dynamic investigation of the surfactant fraction of authentic atmospheric aerosols, using this new extraction method and samples collected in Grenoble, France, from June 2009 to January 2010 (ref. 16 ). The results reveal the existence of adsorption barriers to the surfactant concentration gradients, affecting their equilibration time. These aspects have been overlooked in the theoretical and instrumental investigations of cloud activation until now, which might have limited the understanding of these processes. Delayed equilibrium and adsorption barrier This first section presents the time-dependent surface tension curves ( σ versus t , where t is time in s) obtained in this work, and their implications for the kinetic regime (apparent diffusion coefficient) and molecular interactions affecting the surfactants. The time-dependent curves are presented in Fig. 1 , each point containing about ±10% of uncertainties, mostly because of the variability between measurements (see Methods). Note that the equilibrium curves ( σ eq versus C, where C is the bulk concentration of surfactant) for the atmospheric samples studied in this work have been presented elsewhere [16] . All the curves in Fig. 1 reach their minimum after substantial delays: 15 s–5 min for the aerosol extracts, about 15 s for rhamnolipid and surfactin, and 2–90 min for sodium dodecyl sulphate (SDS). These curves were compared with a model identifying distinct kinetic regimes [19] during this long equilibration, as illustrated in Fig. 1a : a rapid fall (I) from the pure water value (72.8 mN m −1 ) to σ o , too fast to be captured by our instrument; a meso-equilibrium (II) characterized by a time, t m , and during which the surface tension decreases to σ m ; and finally the equilibrium region (III) where the minimum, σ eq , is ultimately reached. 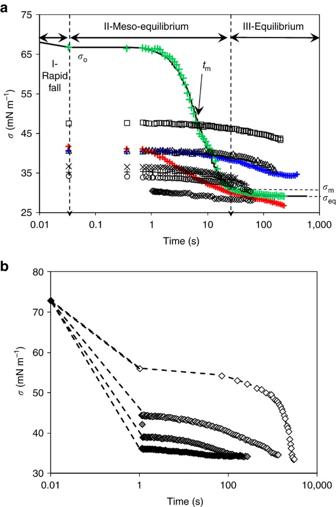Figure 1: Dynamic surface tension curves for the aerosol samples and reference compounds. (a) Curves obtained for surfactin (green), rhamnolipids (red) and SDS (blue), and the aerosol samples (black symbols): 4 June 2009 (diamonds), 7 July 2007 (circles), 16 July 2009 (pluses), 10 November 2009 (crosses), 20 November 2009 (squares) and 3 January 2010 (triangles) in water. (b) Curves obtained by adding increasing amounts of NaCl to SDS solutions, 3.4 mM: no salt (white symbols), +4.2 mM NaCl (pale grey), +8.4 mM NaCl (darl grey) and +12.6 mM NaCl (black). This model was applied to the experimental curves by fitting the following equation [19] : Figure 1: Dynamic surface tension curves for the aerosol samples and reference compounds. ( a ) Curves obtained for surfactin (green), rhamnolipids (red) and SDS (blue), and the aerosol samples (black symbols): 4 June 2009 (diamonds), 7 July 2007 (circles), 16 July 2009 (pluses), 10 November 2009 (crosses), 20 November 2009 (squares) and 3 January 2010 (triangles) in water. ( b ) Curves obtained by adding increasing amounts of NaCl to SDS solutions, 3.4 mM: no salt (white symbols), +4.2 mM NaCl (pale grey), +8.4 mM NaCl (darl grey) and +12.6 mM NaCl (black). Full size image Note that equation (1) involves σ m , but not σ eq , that is difficult to determine experimentally (small variations of σ over long timescales). Reliable fits to the model were obtained for all the experimental curves, even for those not completely reaching equilibrium because the parameters in equation (1) are fairly independent. In particular, the aerosol extracts corresponded to σ o =30–48 mN m −1 , σ m =28–42 mN m −1 and n =0.95–1.5. The values obtained for the characteristic time of the meso-equilibrium, t m , are given in Table 1 and contain about ±10% of uncertainties. Among the different regimes identified by the model and equation (1), while the rapid fall results in a substantial and almost instantaneous decrease of the surface tension, the meso-equilibrium appears to be responsible for most of the delay to equilibration, the overall equilibration time, t eq , being of the order of 2 × t m . Table 1 List of the samples studied and results of this work. Full size table Similar delays to equilibration and kinetic regimes have been evidenced for many surfactants in the literature and shown to result from molecular processes much slower than diffusion and kinetically limiting [19] , [20] , [21] , [22] , [23] . To confirm that this is also the case for the aerosol surfactants studied in this work, their apparent diffusion coefficients, D a (cm 2 s −1 ), were determined using the following equation [23] : where R is the gas constant, T is the temperature, slope is the initial slope of the curves when plotted against 1/ t 1/2 (that is, d σ /d t −1/2 ) and Γ is the surface excess concentration of surfactant molecules. The bulk concentration, C , for the reference surfactants was assumed to be equal to their average concentration in solution. For the aerosol extracts, C was not known but estimated from their equilibrium curves reported in the study by Baduel et al . [16] On these curves, the critical micelle concentration (CMC), located at the bottom of the rapid transition, is reached after diluting the initial extract by about a factor 3 (from 40 to 120 μl). C was thus estimated to be about 3 × CMC in these samples, which, assuming CMC ~50 μM (20–84 μM for C 13 –C 15 surfactins [24] and ~10 μM for rhamnolipids [25] ) gave C ~150 μM in the atmospheric extracts. The surface excess concentration Γ was then calculated from the derivative of the equilibrium surface tension curves ( σ eq versus C ) at C =CMC (that is, at its maximum), according to the Gibbs equation [17] , [23] : The values of Γ thus obtained are given in Table 1 . For rhamnolipids and surfactin they are within 10% of those reported in the literature [17] , [18] , but for the atmospheric samples they are estimated to contain ~20% uncertainties because of the uncertainties on the equilibrium curves ( σ eq versus C ) reported in Baduel et al . [16] The apparent diffusion coefficients, D a , thus obtained from equation (2) are given in Table 1 . They are much smaller, in most cases by more than one order of magnitude, than actual diffusion coefficients for surfactants, which are typically of the order of 2–7 × 10 −6 cm 2 s −1 (ref. 26 ). This confirms that the aerosol surfactants studied in this work are kinetically limited by molecular processes much slower than diffusion. Note that, as discussed below, the classical Gibbs equation (3) is likely to overestimate the surface/bulk ratio, and therefore Γ , but more realistic values would give even smaller diffusion coefficients. Interestingly, the diffusion coefficients determined in previous works for humic-like substances using a similar approach showed that these compounds were limited by diffusion [6] . Slow molecular regimes such as those identified for the aerosol surfactant fractions in this work have been shown in the literature to be caused by adsorption barriers at the air–water interface, keeping the surfactant molecules below this interface. Depending on the surfactant, these barriers can be of different nature: electrostatic interactions for ionic surfactants [27] , [28] , micellization or lamellization processes [17] , [29] , [30] , or impurities (the later especially for SDS) [31] . Dynamic surface tension curves similar to those obtained in this work have thus been accounted for by adding electrostatic terms [27] , micellization or lamellization terms [30] , to the classical Gibbs equation. As a result, the surfactant surface/bulk concentration gradients obtained were much less pronounced than those given by the classical equation, thus by partitioning models. Such small gradients have been confirmed experimentally by ion scattering [32] and angle resolved X-ray photoelectron [33] , [34] spectroscopies, which have observed surface/bulk concentration ratios between 2 and 8. These ratios will be compared with those predicted by partitioning models in the Discussion section. Effects of concentration and salt on the meso-equilibrium This section investigates the parameters affecting the characteristic time of the meso-equilibrium, t m , as the later appears to limit the equilibration time of surfactants. The surfactant concentration, C , is known to affect the adsorption barriers described above because surfactant molecules screen off the electrostatic interactions at the air–water interface and/or, at large concentration, accelerate micellization [17] , [19] , [27] , [28] . The variation of t m with C was investigated in this work by diluting each aerosol extract 10–15 times and measuring the dynamic surface tension each time ( Fig. 2 ). The time-dependent curves obtained were then fitted with equation (1) to determine t m . 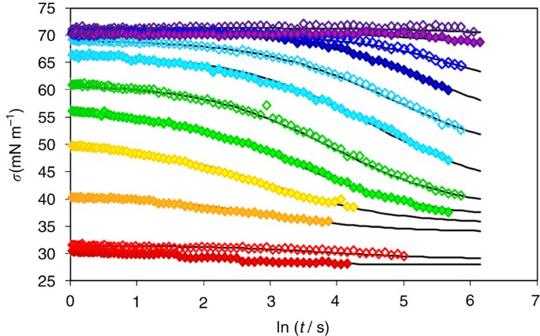Figure 2: Effect of surfactant concentration on the dynamic curves. Dynamic curves obtained by progressively diluting the aerosol surfactant extract of 04 June 2009 and fit to equation (1) (lines) to determinetmfor each concentration. From bottom: pure extract (filled red symbols), and dilutions by 0.67 (open red symbols), 0.44 (orange), 0.33 (yellow), 0.24 (filled green), 0.15 (open green), 0.095 (filled cyan), 0.065 (open cyan), 0.044 (filled blue), 0.028 (open blue), 0.017 (filled purple) and 0.009 (open purple). This quantity was found to vary inversely with the relative concentration of surfactant (or dilution factor), Figure 2: Effect of surfactant concentration on the dynamic curves. Dynamic curves obtained by progressively diluting the aerosol surfactant extract of 04 June 2009 and fit to equation (1) (lines) to determine t m for each concentration. From bottom: pure extract (filled red symbols), and dilutions by 0.67 (open red symbols), 0.44 (orange), 0.33 (yellow), 0.24 (filled green), 0.15 (open green), 0.095 (filled cyan), 0.065 (open cyan), 0.044 (filled blue), 0.028 (open blue), 0.017 (filled purple) and 0.009 (open purple). Full size image with n =0.86–2.38 ( Fig. 3 ). These results are consistent with the value of n =1.7 reported for C 15 -Surfactin [17] , and n =1.88 and 2.04 for a series of C 8 –C 12 surfactants [21] . 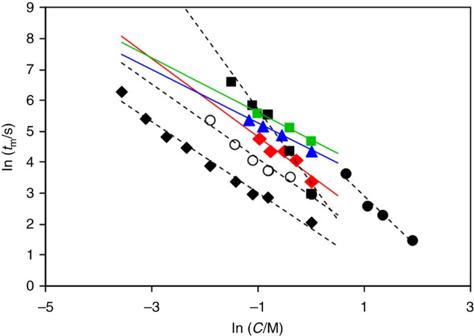Figure 3: Variations of the meso-equilibrium with surfactant concentration. Variations of the characteristic time of the meso-equilibrium,tm, with the relative concentration of surfactant for the different aerosol samples, and best fits (lines): 04 June 2009 black diamonds (n=1.15), 07 July 2009 red diamonds (n=1.26), 17 July 2009 white circles (n=1.20), 10 November 2009 black squares (n=2.38), 20 November 2009 blue triangles (n=0.86) and 03 January 2010 green squares (n=0.87). Comparison with data for C15 surfactin from the study by Razafindralamboet al.17(black circles,n=1.7). Figure 3: Variations of the meso-equilibrium with surfactant concentration. Variations of the characteristic time of the meso-equilibrium, t m , with the relative concentration of surfactant for the different aerosol samples, and best fits (lines): 04 June 2009 black diamonds ( n =1.15), 07 July 2009 red diamonds ( n =1.26), 17 July 2009 white circles ( n =1.20), 10 November 2009 black squares ( n =2.38), 20 November 2009 blue triangles ( n =0.86) and 03 January 2010 green squares ( n =0.87). Comparison with data for C15 surfactin from the study by Razafindralambo et al . [17] (black circles, n =1.7). Full size image Another known parameter affecting the dynamic behaviour of surfactants is the presence of large amounts of salt, in particular of sodium chloride (NaCl) [19] , [21] , [23] , [27] , [28] . This salt is known to markedly reduce the equilibration time of surfactants by screening off the electrostatic barriers to adsorption much more efficiently than surfactant molecules, whereas not affecting the CMC or σ eq (ref. 18 ). The effect of adding NaCl on the equilibration time of surfactant was thus investigated in this work but only with the reference surfactants, as the atmospheric extracts had been entirely used for the dilution study. The dynamic surface tension curves obtained by progressively increasing the concentrations of NaCl reached their equilibrium correspondingly faster, as illustrated in Fig. 1b for SDS. By fitting these curves with equation (1) smaller values of t m than in the absence of salt were also obtained ( Table 1 ), although this was less obvious for rhamnolipid and surfactin than for SDS, because of the large uncertainties in locating the meso-equilibrium on these curves. The apparent diffusion coefficient D a was also determined for these salt mixtures, assuming an increase of Γ by a factor 2 for [NaCl] >30 mM (ref. 18 ). The results are given in Table 1 , where it can be seen that D a increases with NaCl concentration, the diffusion regime being reached for [NaCl] ≥0.04–0.1 M. These results confirm both the existence of adsorption barriers and the efficiency of NaCl in suppressing them at large concentration. Adding large amounts of salt to surfactants could thus be used in laboratory to diagnose potential time limitations of the instruments (see Discussion). The surface/bulk ratios resulting from the adsorption barriers on surfactants will now be compared with the predictions of partitioning models. These models take into account the large surface/bulk ratios of surfactants to calculate smaller bulk concentrations, resulting in small Raoult’s terms. These small Raoult’s terms cancel out the surface tension effect and strongly reduce the expected cloud-forming efficiency of these compounds [8] . Surface/bulk number ratios, n s / n b , predicted by partitioning models are in the range of 10–20 (refs 8 , 10 ). For a particle with a radius of 300 nm and a surface layer of 3 nm, for instance, a number ratio of 11 corresponds to a concentration ratio of 352. The concentration ratios of 2–8 measured experimentally for surfactants [32] , [33] , [34] thus indicate that those calculated by the partitioning models are overestimated by a factor 100 in average (44–176), and the corresponding values of n b are underestimated by the same factor. The Raoult’s term should thus be also underestimated by about 100, as it is proportional to n b , which should substantially underestimate the cloud-forming efficiency of surfactants. In addition to these thermodynamic considerations, the implications of this work for the equilibration timescale of surfactants in atmospheric particles will now be discussed. First, we will determine whether the decrease of the surface tension during the rapid fall is sufficient to induce particle activation or if the decrease occurring during the meso-equilibrium is also necessary, in which case the activation timescale would be limited by the meso-equilibrium. For this, time-dependent Köhler curves were calculated for a representative sample (04 June 2009) and taking into account the time variations of σ . These curves were calculated point by point using the same approach as shown in the study by Ekström et al . [15] , [35] and from the Köhler equation: [1] where d is the diameter of the particle, S ( d ) the corresponding supersaturation, a w the activity of water corresponding to the Raoult’s term. The other terms, A , R , and T were all constant. σ was replaced in equation (5) by the time-dependent expression (equation (1)) obtained by fitting the experimental curve for the sample of 04 June 2009. The Raoult’s term, a w , was obtained from osmometric measurements [15] , [35] , [36] . As such measurements could not be made with the samples studied in this work, those made previously with rhamnolipid [15] , which had the most similar properties, were used: According to Kiss and Hansson [36] , the Raoult’s term was then calculated as: where M w is the molar weight of water (18 g l −1 ). The Köhler curves were then calculated for an initial dry particle of diameter of 110 nm. The surfactant concentration in this particle was estimated to be about three times the one in the aerosol extracts, based on the volume ratios of the particulate matter on filters (<10 μl) over those of the extracts (30–40 μl) [15] , [16] . The surfactant concentration in the dry particle was thus assumed to be C ~10 × CMC=5 × 10 −4 M. The Köhler curves obtained for different times between the rapid fall (0.03 s) and equilibrium (here taken at t =10,000 s) are shown in Fig. 4 . These curves evidence a large relative decrease in critical supersaturation, of nearly 30% in relative humidity, occurring after the rapid fall, thus during the meso-equilibrium. This is because, as illustrated in Fig. 2 , while at large surfactant concentrations ( C >CMC) the rapid fall brings σ down to 80 or 90% of the equilibrium value, σ eq , for intermediate concentrations ( C ~0.2–0.5 × CMC) σ o remains at least 20 mN m −1 above this equilibrium. In that case, the additional decrease of σ during the meso-equilibrium is essential to reach activation. For the aerosol samples studied in this work, the critical radius corresponded to this intermediate range of concentration. Their equilibration timescale in sub-micron atmospheric particles, t eq , is therefore limited by the meso-equilibrium. 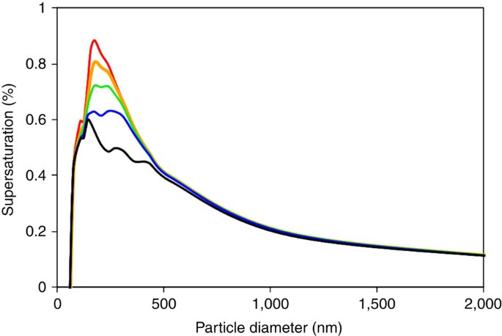Figure 4: Time-dependent Köhler curves. Köhler curves illustrating the effects of the dynamic surface tension on droplet activation for the sample of 04 June 2009:t=0.03 s (just after the rapid fall, red) 10 s (orange), 30 s (green), 100 s (blue) andteq(black). Figure 4: Time-dependent Köhler curves. Köhler curves illustrating the effects of the dynamic surface tension on droplet activation for the sample of 04 June 2009: t =0.03 s (just after the rapid fall, red) 10 s (orange), 30 s (green), 100 s (blue) and t eq (black). Full size image This surfactant equilibration timescale in sub-micron atmospheric particles, t eq , will now be estimated, assuming t eq ~2 × t m and using the variations of t m with different parameters identified in this work. In particular, the variations of t m with the bulk concentration, C , will be assumed to follow equation (4) and other, unknown, parameters will be taken into account empirically as an apparent diffusion coefficient, D a : Combining this expression with equation (4) gives: However, D a also varies with C , which is not taken into account by equation (4), as t m and D a are measured over different kinetic regimes (regions (II) and (III), respectively). Equation (2) indicates an explicit variation of D a with C , but both the slope d σ /d t −1/2 and the surface excess Γ vary with C . d σ /d t −1/2 is expected to increase with C because larger concentrations of surfactants screen off the electrostatic barriers to adsorption. For the dilution series presented above, d σ /d t −1/2 was found to increase linearly with C , thus compensating the explicit C term in the lower hand side of equation (2). However, below the CMC, Γ also increases with C and its variations were determined by assuming that the equilibrium surface tension follows a Syszkowski–Langmuir equation [2] : where σ w , b , a and T are constants. Thus, d σ /dln C and Γ were found to be proportional to C , and D a to C 4 . Combining this expression with equation (9) gave an overall expression for t m : Equation (11) implies that the equilibration time for surfactants in an activated particle, t eq , can be estimated from those measured on large droplets in this work simply by scaling the radius of the droplets and the concentration of surfactant: where the index ‘activ’ relates to the atmospheric droplet and ‘lab’ to the laboratory results obtained in this work. The droplets studied in laboratory had a diameter of 0.8 mm (see Methods), which, to our knowledge, is about the smallest size for which direct surface tension measurement is currently possible. The activated particle will be assumed to be produced from a dry particle of 110 nm of diameter and to reach a critical diameter of about 400 nm. Although this is larger than the critical diameters of the curves in Fig. 4 , it corresponds to those determined previously for rhamnolipids and surfactin [12] , and thus probably more realistic. The growth of the particle from the dry to the critical radius thus corresponds to a volume change of ~48. The corresponding surfactant concentration in the critical particle would thus be 0.2 × CMC, which, according to the curves in Baduel et al . [16] , still corresponds to a significant surface tension reduction ( σ <50 mN m −1 ). Combining the variations in radius and in concentration in equation (11) gave t eq =36–495 s for atmospheric surfactants in activated atmospheric particles ( Table 1 ). For the reference surfactants, the same calculation was made but using the experimental concentrations for C lab , which were between 0.4 × CMC (for SDS 3.4 mM) and 4.9 × CMC (for rhamnolipid). The extrapolation gave t eq =0.1–450 s in activated particles. These results confirm the importance of surfactants for the formation of clouds with slow vertical updraught (~0.1 m s −1 ) such as low clouds or stratus cloud. The equilibration times for aerosol surfactants estimated above are well within the activation times for such clouds, which are between 1 and 30 min, implying that they would have time to reach equilibration and thus fully contribute to cloud droplet formation. The presence of salt in atmospheric particles would further increase their cloud-forming efficiency: in moderate concentrations it would not accelerate surfactant equilibration but increase the Raoult’s term of the particles. But if the salt concentration in some particles, for instance marine aerosols, exceeds a few M the activated particles might still contain 0.04–0.1 M of salt, for which the surfactants reach equilibrium instantly, thus further increasing the cloud-forming potential. However, the equilibration times estimated above for surfactant in atmospheric particles are larger than the residence time of most HTDMA and CCNC instruments, which are typically between 0 and 15 s. This implies that the effects of most surfactants on cloud activation would be beyond the detection of most instruments and would have been largely overlooked until now. Such instrumental limits need now to be further investigated, as they would mask important processes for cloud activation and prevent its understanding. A number of recent observations support the existence of such instrumental limits. First, a comparison between different HTDMAs measuring the same aerosol reported that the cloud-forming efficiency measured by each instrument (in that case as a growth factor) was directly proportional to their operating residence time (0–15 s) [3] . Both the short time differences between these results and the fact that they differ for the same aerosol clearly evidences instrumental limitations on the measurements. Regardless of their origin, such time limitation, effective over <20 s, should largely preclude the observation of surfactant effects. Another argument supporting a time limitation on HTDMA measurements is the contrast between the absence of contribution of surface-active compounds to cloud activation reported for years by short-residence-time HTDMAs ( t <20 s) [37] and the clear involvement of low surface tension aerosols (<50 mN m −1 ) reported recently with longer-residence-time instruments (~50 s) in different regions of the atmosphere [12] , [13] . Although the later observations were dismissed as unphysical by their authors, the present work can reconcile them with theory and underlines the value of such long-residence-time measurements. Finally, series of CCNC experiments combined with surface tension measurements have confirmed both the role of surfactants on cloud activation and the potential existence of instrumental limits bypassed by large concentrations of salt. Not only these works have evidenced an increase of particle activation caused by surface-active compounds but they reported that these effects were strongly enhanced [7] or only observed [14] in the presence of large concentration of salts. Interestingly, very recent works [38] report surfactant effects in the CCN measurements of particles containing large amounts of ammonium sulphate, suggesting that this salt could have a similar effect on surfactant equilibration to NaCl. This work underlines the importance of using alternative approaches to CCNCs and HTDMAs to complete the understanding of cloud activation in the atmosphere. Further investigating the potential instrumental and theoretical limitations identified in this work should now be a priority, and could be achieved either by modifying the current instruments or by developing new techniques. Exploring these long-ignored aspects could open new perspectives on the role of surfactants and their sources on cloud formation in the atmosphere. Aerosol samples and extraction The aerosol samples used in this work were PM 10 fractions (particle diameter <10 μm) collected at the urban site of Grenoble les Frênes (5′74 E; 45′16 N) from June 2009 to January 2010. Each sample was collected over 24 h on 150-mm quartz filters (Pallflex Tissuqartz) previously baked for 2 h at 600 °C. The sampling was made with a high-volume sampler (DIGITEL DA80) operating at 30 m 3 h −1 . The surfactant fraction of these samples was extracted with the method published previously [15] , [16] . The procedure involves three steps as follows: (1) extraction of the filter samples in water; (2) extraction of the surfactants from the water extracts onto silicon tubes for 12 h; and (3) recovery of the compounds from the silicon tubes with methanol, evaporation of the solvent and re-dissolution in water (30–40 μl). After applying this procedure, the complete extraction of all surfactant material from the samples was confirmed by verifying that, after extraction, the surface tension of the solutions were, within uncertainties, the one of pure water (72.8±0.4 mN m −1 ). Dynamic surface tension measurements The dynamic surface tension was studied by the hanging droplet method using a FTÅ 125 tensiometer. The surface tension was determined by comparing the shape of the drop hanging from a syringe to the Young–Laplace equation. A capillary tip of 0.71 mm outside diameter was used, producing drops of a diameter of 0.8 mm. This is about the smallest drop size on which direct surface tension measurements can be performed as, for smaller sizes, the drop shape is not affected enough by the surface tension. The measurements were carried out at 295 K and the tensiometer was calibrated with Milli-Q water. The time resolution of this technique was ~0.03 s and the uncertainties on each surface tension measurement are ~0.4 mN m −1 . Each dynamic surface tension curve was measured three times and the measurements displayed ±10% of variation. These dynamic surface tension measurements lasted about 10–15 min with the atmospheric samples and most reference compounds. Only with SDS it was necessary to perform these measurements over longer timescales (≤1 h). Along with the surface tension, each measurement also provided a real-time monitoring of the droplet volume, thus allowing to check for evaporation. No significant evaporation was observed during the experiments. Chemicals SDS ≥99%, Fluka was used without further purification; C15-Surfactin (MW=1,036.34), ≥98%, Aldrich. Rhamnolipid mixture JBR425 (mono- and di-rhamnolipids), Jeneil Biosurfactant Company, USA, main MW=504.330 g mol −1 (ref. 15 ). NaCl ≥99.6%, Analar Normapur. How to cite this article: Nozière, B. et al . The dynamic surface tension of atmospheric aerosol surfactants reveals new aspects of cloud activation. Nat. Commun. 5:3335 doi: 10.1038/ncomms4335 (2014).